CCN1 is an opsonin for bacterial clearance and a direct activator of Toll-like receptor signaling Expression of the matricellular protein CCN1 (CYR61) is associated with inflammation and is required for successful wound repair. Here, we show that CCN1 binds bacterial pathogen-associated molecular patterns including peptidoglycans of Gram-positive bacteria and lipopolysaccharides of Gram-negative bacteria. CCN1 opsonizes methicillin-resistant Staphylococcus aureus (MRSA) and Pseudomonas aeruginosa and accelerates their removal by phagocytosis and increased production of bactericidal reactive oxygen species in macrophages through the engagement of integrin α v β 3 . Mice with myeloid-specific Ccn1 deletion and knock-in mice expressing CCN1 unable to bind α v β 3 are more susceptible to infection by S. aureus or P. aeruginosa , resulting in increased mortality and organ colonization. Furthermore, CCN1 binds directly to TLR2 and TLR4 to activate MyD88-dependent signaling, cytokine expression and neutrophil mobilization. CCN1 is therefore a pattern recognition receptor that opsonizes bacteria for clearance and functions as a damage-associated molecular pattern to activate inflammatory responses, activities that contribute to wound healing and tissue repair. The rapid emergence of antibiotic-resistant bacteria poses a serious threat to public health globally [1] . Despite the remarkable success of antibiotics in treating bacterial infections since the 1940s, resistance to virtually all available antibiotics has been observed in recent decades. Antibiotic-resistant bacterial infections account for nearly 3 million clinical cases and >35,000 deaths annually in the United States alone [2] , and >700,000 deaths worldwide [3] . Among the most encountered pathogens are the Gram-positive Staphylococcus aureus ( S. aureus ) and the Gram-negative Pseudomonas aeruginosa ( P. aeruginosa ). These bacteria quickly acquire antibiotic resistance, largely through mobile genetic elements such as plasmids and transposons [4] . Methicillin-resistant S. aureus (MRSA) alone accounts for a large portion of nosocomial [5] and community-acquired infections [6] and is a leading cause of endocarditis, septicemia, and skin and soft-tissue infections (SSTIs) [7] , [8] . P. aeruginosa is an opportunistic pathogen commonly found in ventilator-associated pneumonia, catheter-associated urinary tract infections, burn wounds, and blood infections [9] . Although vaccines are under development for these pathogens, none have achieved clinical efficacy to date [10] , [11] . Therefore, there is an urgent need to identify effective therapeutic strategies for such antibiotic-resistant pathogens as S. aureus and P. aeruginosa . Upon bacterial infection, vertebrate hosts mount an onslaught of attacks at the invaders, including activation of the complement system that targets bacteria for lysis or phagocytosis. In addition, resident macrophages that patrol the tissues eliminate microbes by phagocytosis, whereupon the activated macrophages produce cytokines and chemokines to induce inflammation and to recruit immune cells that reinforce bacterial removal and initiate adaptive immunity [12] . Accordingly, defects in phagocytes lead to impaired host defense against infections [13] . Bacterial pathogens are typically detected by host proteins known as pattern recognition receptors (PRRs) that recognize and bind distinct microbial components, or pathogen-associated molecular patterns (PAMPs) [14] . Among the best characterized PRRs are cell surface Toll-like receptors (TLRs), which are potent activators of inflammatory responses upon recognition of PAMPs [15] , [16] . TLRs can also mediate sterile inflammation by interacting with damage-associated molecular patterns (DAMPs), endogenous danger molecules that are released from damaged or dying cells [17] , [18] . Professional phagocytes express PRRs that bind PAMPs and induce phagocytosis directly, such as macrophage mannose receptor and macrophage scavenger receptors [19] , [20] , as well as opsonins that recognize PAMPs and connect the bacteria to phagocytes for elimination [21] , [22] . As these mechanisms of host defenses are unrelated to the bactericidal pathways of antibiotics, treatments that stimulate or enhance these host defenses may provide therapeutic strategies for the clearance of microbial pathogens irrespective of their antibiotic resistance status. Ccn1 ( Cyr61 ) encodes a 40 kDa matricellular protein that is essential for embryonic development [23] , [24] . In adults, Ccn1 expression is associated with inflammation and is required for successful injury repair in the skin [25] , [26] , liver [27] , and gut [28] . Structurally, CCN1 is organized into four conserved domains with homologies to insulin-like growth factor-binding protein (IGFBP), von Willebrand factor type C repeat (vWC), thrombospondin type-1 repeat (TSR), and a cysteine-knot motif in the C-terminal (CT) domain (Supplementary Fig. 1 ) [29] . Mechanistically, CCN1 acts through direct binding to specific integrin receptors in a cell type-specific manner, engaging coreceptors in some contexts [30] , [31] . The specific CCN1-binding sites for several integrin receptors, including α v β 3 /α v β 5 , α 6 β 1 , and α M β 2 , have been identified [29] , [30] . We have recently shown that CCN1 promotes efferocytosis, or phagocytosis of apoptotic cells, by binding phosphatidylserine, the “eat-me” signal on apoptotic cells and bridging them to macrophages for elimination through engagement of the phagocytic receptor, integrin α v β 3 [25] . Consequently, CCN1 stimulates the removal of apoptotic neutrophils and accelerates wound healing progression. Here, we have found that CCN1 functions as an opsonin for bacterial clearance through specific binding to PAMPs of S. aureus and P. aeruginosa , inducing their phagocytic elimination through engagement of integrin α v β 3 on phagocytes. Additionally, CCN1 enhances bacterial killing in macrophages by increasing the production of bactericidal reactive oxygen species (ROS). Independent of its opsonin activity, CCN1 can also directly bind and activate TLR2 and TLR4 to induce the expression of proinflammatory cytokines in a MyD88-dependent manner. Altogether, these results show that CCN1 is a PRR that induces opsonophagocytosis of bacteria and a DAMP that can trigger sterile inflammation through activating TLR signaling. CCN1 binds S. aureus and P. aeruginosa through PAMPs Based on the finding that CCN1 induces efferocytosis of apoptotic neutrophils [25] , we investigated the possibility that CCN1 may also target bacterial pathogens for removal by phagocytosis, an activity that requires specific recognition of bacterial PAMPs. Thus, we first assessed whether CCN1 can recognize and bind the Gram-positive S. aureus and the Gram-negative P. aeruginosa in a solid-phase-binding assay. Indeed, S. aureus showed efficient binding to immobilized CCN1, with half-maximal binding occurring at ~10 pmol per well CCN1 (Fig. 1a ). Soluble CCN1 also bound S. aureus efficiently as observed by flow cytometry (Supplementary Fig. 2 ). S. aureus can bind various host extracellular matrix (ECM) proteins by expressing bacterial adhesins, including the fibronectin-binding protein (FnBP) [32] , although the specific S. aureus strain (MRSA USA300) used in this study does not express the collagen adhesin (Cna) [33] . Consistently, S. aureus bound immobilized fibronectin (FN) in a dose-dependent manner with half-maximal binding at ~20 pmol per well but failed to bind collagen I (Col1α1; Fig. 1a ). Both the CCN1-D125A mutant protein [34] , which is unable to bind integrins α v β 3 /α v β 5 as a result of a single amino acid substitution (Asp125 to Ala), and the CCN1-DM mutant [35] , which is defective for binding integrins α 6 β 1 /α M β 2 , were able to bind S. aureus with affinities similar to that of wild type (WT) CCN1 (Fig. 1b ). Thus, the CCN1-binding site(s) for S. aureus are distinct from those for integrins α v β 3 /α v β 5 and α 6 β 1 /α M β 2 . Fig. 1: CCN1 binds S. aureus and P. aeruginosa through PGN and LPS, respectively. CCN1 binding to S. aureus ( a–c ) and P. aeruginosa ( d–f ) was evaluated using a solid-phase-binding assay. a S. aureus bound to surfaces coated with CCN1-WT or other ECM proteins (FN fibronectin, LN laminin, Col1α1 collagen type I) was quantified using polyclonal anti- S. aureus antibodies. CCN1 and FN bound to S. aureus , whereas LN and Col1α1did not. b Binding assay of S. aureus to recombinant CCN1-WT, CCN1-D125A, and CCN1-DM proteins as above. c Binding of S. aureus to CCN1 deletion mutant proteins as above. d Solid-phase-binding assays for P. aeruginosa were performed as above and detected with polyclonal anti- P. aeruginosa antibodies. e Binding assay showing P. aeruginosa binding to CCN1-WT and CCN1-D125A, but not CCN1-DM. f Solid-phase-binding assays with CCN1 deletion mutants. All assays were done in triplicates and data are expressed as mean ± s.d. Statistical evaluation was performed by one-sided, two-sample with equal variance t -tests. ** p < 0.01, n.s. = not significant. g Bacterial molecular patterns (PGN of S. aureus ; LTA of S. aureus ; LPS of P. aeruginosa ; 1 µg each) and BSA as control spotted on nitrocellulose membranes were incubated with CCN1 proteins (WT, D125A, or DM; 2 µg each in PBS) and bound CCN1 was visualized using anti-CCN1 antibodies. Dot blot shown is a representative image. h Senograms of SPR analysis of CCN1 binding to LPS. CCN1 at various concentrations was used as analyte to detect binding to LPS immobilized on HPA hydrophobic sensor chip. K a , K d , and K D values were obtained by kinetic analysis. Full size image We endeavored to identify the region of CCN1 responsible for binding S. aureus using a series of deletion mutants (Supplementary Fig. 1 ). Mutants that contain the TSR domain (ΔCT and TSR alone) showed as strong binding to S. aureus as CCN1-WT, whereas mutants containing the vWC domain (IGFBP-vWC and vWC alone) displayed strong to moderate binding (Fig. 1c ). However, the IGFBP domain alone did not bind S. aureus . These results suggest that CCN1 binds S. aureus through the TSR and vWC domains, whereas the CT domain is dispensable (Fig. 1c ). Prominent among PAMPs of Gram-positive bacteria are the cell wall components peptidoglycan (PGN) and lipoteichoic acid (LTA). We found that CCN1 proteins (WT, D125A, or DM) bound to immobilized PGN, but not LTA (Fig. 1g ). Immunoblotting also showed that both the vWC and TSR domains could bind PGN individually, but not the IGFBP domain (Supplementary Fig. 3 ). These results demonstrate that CCN1 directly binds S. aureus through its vWC and TSR domains by recognizing PGN, a bacterial PAMP. CCN1 also exhibited strong binding to P. aeruginosa in a dose-dependent manner, with half-maximal binding at ~20 pmol per well CCN1 (Fig. 1d ). Other ECM proteins, including FN, LN, and Col1α1, did not show binding (Fig. 1d ). Remarkably, whereas CCN1-WT and CCN1-D125A bound P. aeruginosa with similar dose-dependence, CCN1-DM was completely unable to bind, indicating that the essential binding site for P. aeruginosa was disrupted in CCN1-DM (Fig. 1e ). Consistently, all deletion mutants lacking the CT domain tested (ΔCT, IGFBP-vWC, IGFBP) failed to bind P. aeruginosa (Fig. 1f ). Mutations in CCN1-DM changed several lysine residues and an arginine to glycines in the CT domain (Supplementary Fig. 1 ), rendering CCN1 unable to bind heparin, a polysaccharide of the glycosaminoglycan family [35] , [36] . Thus, we postulated that CCN1-DM may also be defective for binding lipopolysaccharides (LPS), a PAMP of Gram-negative bacteria. Indeed, both CCN1-WT and CCN1-D125A bound immobilized LPS from P. aeruginosa , but not CCN1-DM (Fig. 1g ). We further performed surface plasmon resonance (SPR) analysis to evaluate the binding of CCN1 to LPS, which was immobilized on an HPA hydrophobic sensor chip (Fig. 1h ). Sensorgrams showed high-affinity CCN1 binding to LPS with a K D of 67.4 nM. CCN1 also bound to the Gram-positive Streptococcus pneumoniae and the Gram-negative Salmonella typhimurium , supporting the notion that CCN1 may bind a broad spectrum of bacterial species through PAMPs (Supplementary Fig. 4 ). These results show that CCN1 is a PRR that can directly recognize and bind bacterial PAMPs, including PGN in Gram-positive bacteria and LPS in Gram-negative bacteria. CCN1 is an opsonin that stimulates phagocytosis of bacteria Given the ability of CCN1 to bind bacterial PAMPs (Fig. 1 ) and to stimulate phagocytosis [25] , we hypothesized that CCN1 may act as an opsonin to stimulate bacterial clearance by phagocytosis. To test this possibility, we incubated bone marrow-derived macrophages (BMDMs; labeled green) with S. aureus bioparticles (pHrodo® conjugates, labeled red). Engulfment of S. aureus by macrophages was observed by fluorescence microscopy within 45 min (Fig. 2a ). The addition of CCN1 protein stimulated engulfment by ~5-fold (Fig. 2a, b ). Inhibition of actin polymerization with cytochalasin D abrogated bacterial uptake, confirming phagocytosis (Supplementary Fig. 5 ). The CCN1-D125A mutant protein failed to enhance phagocytosis, whereas CCN1-DM was fully active (Fig. 2a, b ), indicating that α v integrins are the essential receptors for CCN1-induced phagocytosis. Consistently, dicer-substrate short interfering RNAs (DsiRNA)-mediated knockdown of either integrin α v ( Itgav ) or β 3 ( Itgb3) efficiently blocked CCN1-induced phagocytosis, whereas knockdown of α 6 ( Itga6 ), α M ( Itgam ), or β 2 ( Itgb2 ) did not (Fig. 2c and Supplementary Fig. 6 ). Knockdown of integrin β 5 ( Itgb5 ) only partially inhibited phagocytosis, suggesting that integrin α v β 3 is the primary phagocytic receptor, whereas α v β 5 plays an auxiliary role. Thus, cilengitide, a cyclic-RGD peptide that selectively blocks integrins α v β 3 /α v β 5 , obliterated CCN1-induced phagocytosis (Fig. 2d ). Likewise, CCN1-WT, but not CCN1-D125A, enhanced phagocytic uptake of S. aureus in bone marrow-derived neutrophils (BM-PMNs; Supplementary Fig. 7 ) and in differentiated THP.1 human macrophages (Fig. 2e ), indicating the involvement of the same receptors in CCN1-induced phagocytosis of bacteria in neutrophils and human macrophages. Of note, integrin α M β 2 is also known as CR3 (CD11b/CD18), the type 3 complement receptor that binds iC3b to promote phagocytosis [37] , but is not involved in CCN1-induced phagocytosis based on these mutational (CCN1-DM) and DsiRNA knockdown results. Consistent with previous findings that α v β 3 -mediated phagocytosis requires activation of Rac1 [25] , [38] , inhibition of Rac1 by NSC23766 blocked CCN1-induced phagocytosis (Fig. 2d ). Concordant with the role of PI3K in Rac1-dependent cytoskeletal rearrangement [39] , PI3K inhibitor LY294002 reduced CCN1-induced phagocytosis (~50%), whereas ERK inhibitor (PD98059) or p38 MAPK inhibitor (SB203580) had no effect (Supplementary Fig. 5 ). Furthermore, commercially available CCN1 protein from different cellular sources also bound PGN and LPS and induced cilengitide-inhibitable phagocytosis of S. aureus (Supplementary Fig. 8 ), suggesting that these reproducible functions are bona fide activities of CCN1. Fig. 2: CCN1 stimulates phagocytosis of bacteria through α v integrins in macrophages. BMDMs (labeled with CellTracker TM Green) were pretreated with either BSA, CCN1-WT, CCN1-D125A, or CCN1-DM proteins (2 µg per ml) followed by incubation with bacteria for 45 min. a Phagocytosis of S. aureus (pHrodo Red conjugates) is shown in representative images from fluorescence microscopy. Scale bar = 40 µm. b Quantification of phagocytosis of S. aureus by BMDMs pretreated with various proteins. c BMDMs were transfected with DsiRNAs to knockdown integrins α 6 , α v , β 3 , β 5 , α M , or β 2 ; knockdown efficiencies are shown in Supplementary Fig. 6 . Cells were then pretreated with CCN1 or BSA, and phagocytosis of S. aureus was quantified. NT-1, non-targeting RNA. d Effect of cilengitide (1 µM) and the Rac1 inhibitor NSC23766 (10 µM) on CCN1-induced phagocytosis of S. aureus . e CCN1-induced phagocytosis in differentiated THP.1 human macrophages. f BMDMs were pretreated as above and then incubated with live P. aeruginosa (MOI of 10) for 45 min, followed by gentamycin (200 µg per ml for 15 min) treatment. Phagocytosis was measured by enumeration of bacterial colonies grown from cell lysates. g Effects of DsiRNA-mediated knockdown of integrins α v , β 3 , α M , or β 2 on CCN1-induced phagocytosis of P. aeruginosa . All data are expressed as mean ± s.d. in triplicate determinations. Statistical evaluation was performed by one-sided, two-sample with equal variance t -tests. * p < 0.05, ** p < 0.01, n.s. = not significant. Source data are provided as a Source Data file. Full size image To evaluate whether CCN1 can also induce phagocytosis of Gram-negative bacteria, we tested its effects on P. aeruginosa (Fig. 2f, g ). BMDMs were incubated with P. aeruginosa and phagocytosed bacteria were enumerated after extracellular bacteria were eliminated by gentamycin. We found that CCN1 also enhanced phagocytic uptake of P. aeruginosa , whereas CCN1-D125A was inactive (Fig. 2f ). CCN1-DM, which was fully able to stimulate phagocytosis of S. aureus , was completely unable to enhance phagocytosis of P. aeruginosa (Fig. 2f ). That CCN1-DM was incapable of binding LPS or P. aeruginosa (Fig. 1e, g ) provided a clear explanation for this finding and indicated that binding to bacteria through PAMP is critical for CCN1-induced bacterial clearance. Knockdown of either α v or β 3 blocked CCN1-induced phagocytosis of P. aeruginosa , whereas knockdown of α M or β 2 had little effect (Fig. 1g ). These results show that CCN1 opsonizes both Gram-positive and Gram-negative bacteria for phagocytosis, engaging integrin α v β 3 as the primary phagocytic receptor. CCN1 increases ROS for bacterial killing after phagocytosis Upon phagocytosis, ingested bacteria are trapped in vacuoles, or phagosomes, which undergo maturation to become phagolysosomes with diverse antimicrobial arsenals, including microbicidal peptides, lipases, and capacity to generate reactive oxygen species (ROS) [40] . CCN1 is known to induce ROS production in other biological contexts [26] , [41] , prompting us to test whether CCN1 can facilitate bacterial killing following phagocytosis by inducing ROS. To monitor bacterial killing, we allowed BMDM phagocytosis of S. aureus to proceed for 90 min and eliminated the remaining extracellular bacteria by lysostaphin [42] . BMDMs were then treated with CCN1 and the number of surviving intracellular bacteria was monitored over time. As shown in Fig. 3a , the viable S. aureus count in CCN1-treated BMDMs was significantly lower than that of bovine serum albumin (BSA)-treated control after a 3 h chase period, indicating that CCN1 accelerated bacterial killing after phagocytosis. Fig. 3: CCN1 enhances bacterial killing after phagocytosis through ROS production. a Lysostaphin protection assay for assessing S. aureus killing after phagocytosis. After BMDMs phagocytosed S. aureus and extracellular bacteria were eliminated by lysostaphin, cells were treated with CCN1 or BSA (2 μg per ml each) and viable bacteria inside BMDMs were enumerated at indicated chase periods. b Superoxide ( O 2 − ) was measured by dihydroethidium (DHE, 5 µM) staining in BMDMs treated with recombinant CCN1 proteins (WT, D125A, or DM; 2 µg per ml each) for 30 min. Representative images shown were acquired from fluorescence microscopy. Bar = 40 µm. c High-magnification images were taken from at least ten random fields and mean fluorescence intensity (MFI) was calculated using Image J software. d ROS production was quantified as MFI using DHE fluorescence in BMDMs pretreated with cilengitide (1 μM), followed by CCN1 or BSA (2 µg per ml each). e S. aureus killing assays were performed as in a with cilengitide pretreatment. f The effects of various inhibitors on CCN1-induced ROS production. All inhibitors were added 30 min prior to CCN1 treatment. Rac1 inhibitor NSC23766 (10 µM); NOX inhibitor Apocynin (10 µM); NOX2 inhibitor GSK2795039 (10 µM); NOX1 inhibitor ML-171 (10 µM). g Effects of various inhibitors on bacterial killing using lysostaphin protection assays as above. All data were acquired from at least three independent assays and are expressed as mean ± s.d. in triplicate determinations. Statistical evaluation was performed by one-sided, two-sample with equal variance t -tests. ** p < 0.01, n.s. = not significant. Source data are provided as a Source Data file. Full size image Next, we examined whether CCN1 stimulated ROS production to enhance bacterial killing. Treatment of BMDMs with CCN1-induced ROS production within 30 min as judged by staining with dihydroethidium (DHE), a superoxide ( O 2 − ) detection dye (Fig. 3b, c ). CCN1-DM also induced ROS production but not CCN1-D125A, indicating that CCN1 acts through α v integrins (Fig. 3b, c ). Accordingly, cilengitide effectively abolished CCN1-induced ROS and subsequent bacterial killing (Fig. 3d, e ). In macrophages, NADPH oxidase 2 (NOX2) is the principal enzyme responsible for superoxide production [43] . Whereas Rac1 is an activating subunit of NOX2 in macrophages, Rac2 activates NOX2 in neutrophils [44] , [45] . Consistently, the Rac1 inhibitor NSC23766 blocked CCN1-induced ROS production and bacterial killing (Fig. 3f, g ). Apocynin, a non-isoform-specific NOX inhibitor and a ROS scavenger, exhibited strong inhibitory effects (Fig. 3f, g ). The NOX2 inhibitor (GSK2795039), but not NOX1 inhibitor (ML-171), diminished CCN1-induced ROS production and bacterial killing (Fig. 3f, g ). These results show that CCN1 enhances microbial killing after phagocytosis by the induction of ROS through integrin α v -mediated activation of Rac1-NOX2. CCN1 is critical for bacterial clearance in animal models Given that CCN1 opsonizes bacteria for phagocytosis and killing, we investigated the role of CCN1 in host defense against bacterial infections in animal models. Since professional phagocytes are derived from the myeloid lineage, we generated mice with Ccn1 deleted specifically in myeloid cells by crossing Ccn1 flox/flox mice with the deleter strain LysM-Cre , yielding Ccn1 flox/flox ; LysM-Cre mice (hereafter called Ccn1 ΔMyeloid mice; Supplementary Fig. 9 ). Ccn1 expression in Ccn1 ΔMyeloid mice was greatly reduced in peritoneal macrophages, BMDMs, and BM-PMNs, but remained at WT levels in splenic B and T lymphocytes (Fig. 4a ), indicating Ccn1 deletion specifically in myeloid cells. Fig. 4: Ccn1 expression in myeloid cells is critical for host defense against S. aureus infections. a Ccn1 mRNA in peritoneal macrophages (MΦ), BMDMs and PMNs, and splenic B and T cells from Ccn1 flox/flox and Ccn1 ΔMyeloid mice was analyzed using qRT-PCR. Myeloid-specific deletion was confirmed using splenic B and T cells as controls. Data are represented as mean ± s.d. from triplicate experiments. Statistical evaluation was performed by one-sided, two-sample with equal variance t -tests. * p < 0.05, ** p < 0.01, n.s. = not significant. b Survival of Ccn1 flox/flox ( n = 13) and Ccn1 ΔMyeloid ( n = 12) mice after infection with S. aureus (7.5 × 10 8 CFU per mouse, i.v . ). c Tissue colonization of S. aureus in Ccn1 flox/flox and Ccn1 ΔMyeloid mice infected with S. aureus (2 × 10 8 CFU per mouse, i.v . ). Bacterial counts in liver, kidney, and heart ( n = 8 each) 5 days post infection were evaluated by growth of serially diluted tissue homogenates on tryptic soy agar with 5% sheep blood and plotted as CFU per mg tissues. d Histological examination of liver and kidney of Ccn1 flox/flox and Ccn1 ΔMyeloid mice at day 5-post infection. Representative images are shown. H&E staining showed the presence of pyogenic abscesses (arrowheads in left panels) in both liver and kidney from Ccn1 ΔMyeloid mice, whereas no pyogenic abscesses were found in Ccn1 flox/flox mice. Boxed regions with dotted line are expanded in high magnification in middle panels. Asterisk (*) points to nidus, yellow rectangular box indicates pseudo-capsule, and bidirectional arrow shows regions of neutrophils. S. aureus colonization was visualized in adjacent sections using anti- S. aureus antibodies (green, Alexafluor488-anti-rabbit IgG) in immunofluorescence staining (right panels). DAPI (blue) was used as a counterstaining. Scale bar = 100 μm. e Blood dissemination of S. aureus was determined at indicated days after subcutaneous infection of S. aureus (5 × 10 5 CFU in 50 µl PBS) in Ccn1 flox/flox and Ccn1 ΔMyeloid mice ( n = 9 each). Blood (10 µl) was plated for colony quantification. Source data are provided as a Source Data file. Full size image S. aureus is a leading cause of lethal bacteremia [46] , [47] . To examine the functions of CCN1 in bacteremia, Ccn1 flox/flox (control) and Ccn1 ΔMyeloid mice were infected intravenously ( i.v .) with S. aureus (7.5 × 10 8 CFU per mouse; Fig. 4b ). Remarkably, Ccn1 ΔMyeloid mice exhibited 100% mortality within 5 days, whereas 60% of Ccn1 flox/flox mice survived at least 10 days (Fig. 4b ), showing that myeloid expression of Ccn1 strongly protects against S. aureus bacteremia. Bloodstream infection of S. aureus often disseminates to multiple internal organs, including the liver, kidney, and heart [48] . To examine tissue colonization of disseminated bacteria, we used a reduced dose of S. aureus (2 × 10 8 CFU per mouse; i.v .) to minimize mortality (Fig. 4c, d ). The liver and kidney of Ccn1 ΔMyeloid mice displayed higher bacterial burdens (~5-fold) compared to Ccn1 flox/flox mice 5 days post infection (Fig. 4c ), as confirmed by H&E staining and immunohistochemistry (Fig. 4d ). Both liver and kidney sections from Ccn1 ΔMyeloid mice displayed multiple nidi that are surrounded by pseudo-capsules and massive infiltration of neutrophils, characteristics of S. aureus pyogenic abscesses (Fig. 4d ), which were not observed in Ccn1 flox/flox mice. Bacterial colonization was also much more severe in the Ccn1 ΔMyeloid heart, with ~100-fold more bacterial burden compared to controls (Fig. 4c ). As S. aureus is the most prominent cause of SSTI [49] , we also examined blood dissemination in a skin infection model. After a bolus of S. aureus (4 × 10 6 CFU per mouse) was injected subcutaneously into mouse flank skin, blood dissemination was ~2 orders of magnitude higher in Ccn1 ΔMyeloid mice than controls 1 day post infection, and remained high 2 days post infection while bacterial counts in Ccn1 flox/flox mice approached zero (Fig. 4e ). Similarly, Ccn1 ΔMyeloid mice infected with P. aeruginosa showed increased mortality in bacteremia ( i.v . infection) and sustained blood dissemination in peritonitis ( i.p . infection), indicating that CCN1 also defends against infection by Gram-negative bacteria (Supplementary Fig. 10 ). These results show that Ccn1 expression in myeloid cells, including macrophages and neutrophils, plays a crucial role in bacterial clearance in mouse models of infection. CCN1 drives host defense through its α v integrin-binding site To assess the role of α v integrins-mediated CCN1 phagocytic and bactericidal functions in bacterial clearance in vivo, we examined knock-in mice in which the Ccn1 genomic locus is replaced by alleles encoding either CCN1-D125A ( Ccn1 D125A/D125A mice) [25] or CCN1-DM ( Ccn1 DM/DM mice) [26] . Upon i.v . infection with S. aureus (7.5 × 10 8 CFU per mouse), 90% of Ccn1 D125A/D125A mice perished by day 8 post infection, compared to ~20% mortality in either Ccn1 WT/WT or Ccn1 DM/DM mice (Fig. 5a ). These results indicate that CCN1 functions mediated through α v integrins, including induction of phagocytosis and ROS-dependent killing, are critical for bacterial defense in vivo. Assessment of tissue dissemination upon S. aureus infection (2 × 10 8 CFU per mouse; i.v .) showed significantly higher levels of bacterial load in the kidney and heart from Ccn1 D125A/D125A mice 5 days post infection (Fig. 5b ). Interestingly, robust S. aureus colonization was accompanied by extensive tissue damage and loss of glomerular structures in the kidney cortex from Ccn1 D125A/D125A mice, suggesting that integrin α v -mediated CCN1 functions may play additional roles in parenchymal injury repair (Fig. 5c ). Fig. 5: CCN1 functions mediated through its integrin α v -binding site are crucial for host defense. a Survival was monitored in mice infected with S. aureus (7.5 × 10 8 CFU per mouse, i.v . ). Ccn1 WT/WT , n = 9; Ccn1 D125A/D125A , n = 8; Ccn1 DM/DM , n = 10. b Colonization in the kidney and heart was evaluated in mice infected with S. aureus (2.5 × 10 8 CFU per mouse, i.v . ). Bacterial loads were enumerated by serial dilution of tissue homogenates at day 5-post infection in Ccn1 WT/WT ( n = 16 for kidney, n =  8 for heart), Ccn1 D125A/D125A ( n = 16 for kidney, n = 8 for heart), and Ccn1 DM/DM ( n = 6 for kidney, n = 8 for heart) mice. Statistical evaluation was performed by one-sided, two-sample with equal variance t -tests. ** p < 0.01; n.s. = not significant. c Histological evaluation of the kidney cortex after S. aureus infection. Kidney sections from Ccn1 WT/WT and Ccn1 D125A/D125A mice at day 5-post infection were stained with H&E. Glomeruli (yellow arrowheads) and tubules (black arrows) are intact in Ccn1 WT/WT mice, but severely damaged in Ccn1 D125A/D125A mice. Adjacent sections were visualized in immunofluorescence staining with polyclonal anti- S. aureus antibody (green) and counterstained with DAPI (blue). Scale bar = 100 µm. d Treatment of mice with CCN1 protein accelerated bacterial clearance. Ccn1 WT/WT and Ccn1 D125A/D125A mice ( n = 11 per group per genotype) were challenged with acute peritonitis by infection of S. aureus (2 × 10 7 CFU per mouse, i.p . ), followed by i.p . injection of CCN1 protein (5 µg per mouse) or PBS 1 h-post infection. Total blood was drawn at indicated times and 10 µl was plated for colony enumeration. e Ccn1 flox/flox and Ccn1 ΔMyeloid mice ( n = 6 per group per genotype) were infected with S. aureus and bacterial clearance with or without CCN1 treatment was evaluated as above. Source data are provided as a Source Data file. Full size image Exogenous CCN1 accelerates bacterial clearance Given the strong protective role of CCN1 against bacterial infections, we tested whether administration of exogenous CCN1 protein may accelerate bacterial clearance in infected mice. Mice were infected with S. aureus (5 × 10 7 CFU per mouse, i.p .) for 1 h, followed by CCN1 protein injection. Blood dissemination of S. aureus was observed at 3 h post infection in both Ccn1 WT/WT and Ccn1 flox/flox mice and was largely eliminated by 10 h (Fig. 5d, e ). By contrast, high levels of S. aureus in blood were sustained even after 10 h in both Ccn1 D125A/D125A and Ccn1 ΔMyeloid mice (Fig. 5d, e ). Injection of CCN1 (5 µg per mouse, i.p .) greatly reduced S. aureus blood dissemination, virtually eliminating bacterial counts as early as 3 h post infection in both genotypes (Fig. 5d, e ). These results suggest that administration of exogenous CCN1 may have therapeutic value in the treatment of antibiotic-resistant bacterial infections. CCN1 binds and activates TLR2 and TLR4 Macrophages respond to the presence of microbes by engulfment of the invaders and production of cytokines and chemokines, which marshal the infiltration of neutrophils and other immune cells for both innate and adaptive immune defense [12] . Therefore, we examined whether CCN1 may also contribute to host defense through regulating the inflammatory response. We induced acute peritonitis in mice with i.p . infection of S. aureus (5 × 10 7 CFU per mouse) and measured the levels of inflammatory cytokines and chemokines in peritoneal lavage. Upon infection, both cytokines (TNFα and IL6) and chemokines (KC and MCP1) levels were significantly increased in Ccn1 flox/flox mice, whereas this inflammatory response was greatly reduced in Ccn1 ΔMyeloid mice (Fig. 6a–d ). Consistent with decreased KC chemokine levels (Fig. 6c ), complete blood count (CBC) analysis found fewer circulating neutrophils in Ccn1 ΔMyeloid mice following infection (Fig. 6e ). These results show that Ccn1 expressed in myeloid cells plays a key role in the inflammatory response to bacterial infections. Fig. 6: CCN1 is critical for the host inflammatory response upon bacterial infection. a–d Quantification of cytokines and chemokines in the peritoneum in Ccn1 flox/flox or Ccn1 ΔMyeloid mice ( n = 6 per group per genotype) infected with S. aureus (2 × 10 7 CFU per mouse i.p . ). Peritoneal exudates were analyzed by ELISA to quantify the levels of TNFα ( a ) at 30 min and IL6 ( b ), KC ( c ), and MCP1 ( d ) at 2 h post infection. e Neutrophils and lymphocytes contents in blood drawn at 2 h post infection were determined using Advia 120 analyzer. All data are represented as mean ± s.d. acquired in triplicate determinations. Statistical evaluation was performed by one-sided, two-sample with equal variance t -tests. * p < 0.05, ** p < 0.01. Source data are provided as a Source Data file. Full size image To determine how CCN1 may contribute to the inflammatory response, we tested whether CCN1 can by itself induce inflammation without infection. When i.p . injected into uninfected C56BL/6J ( B6 ) mice, both CCN1-WT and the CCN1-D125A mutant elevated the levels of cytokines (TNFα and IL6) in peritoneal exudates and increased neutrophils in circulating blood (Supplementary Fig. 11 ). These results suggest that CCN1 itself, in the absence of infection, can induce sterile inflammation independent of its binding to integrin α v β 3 and activities downstream of integrin signaling. Sterile inflammation is often induced through TLRs recognizing DAMPs, which signal tissue damage [17] , [18] . Thus, we tested the possibility that CCN1 may directly regulate inflammation through TLRs using mice that lack MyD88 ( Myd88 −/− ), a cytoplasmic adaptor molecule that is essential for the signaling of most TLRs [50] . Remarkably, whereas i.p . injected CCN1 elevated the levels of both cytokines (TNFα and IL6) and chemokines (KC and MCP1) in the peritoneal lavage of B6 mice, it failed to do so in Myd88 −/− mice (Fig. 7a–d ). Consistently, CBC analysis showed no increase in blood neutrophils in Myd88 −/− mice upon CCN1 injection (Fig. 7e ). These results indicate that CCN1-induced inflammatory response in vivo is mediated through a MyD88-dependent mechanism, possibly via TLR signaling. To assess the function of CCN1 in an isolated cell system, we treated BMDMs from B6 and Myd88 −/− mice with CCN1. CCN1 elevated both Tnfa and Il6 mRNAs in B6 BMDMs to levels similar to those induced by PGN, but this induction did not occur in BMDMs from Myd88 −/− mice (Fig. 7f ). As expected, induction of Tnfa and Il6 expression by PGN and LPS was completely obliterated in Myd88 −/− BMDMs, since these PAMPs are known to induce inflammatory genes through TLRs (Fig. 7f ). Likewise, CCN1 also induced inflammatory gene expression in differentiated THP.1 human macrophages (Supplementary Fig. 12 ). Fig. 7: CCN1 induces Myd88 -dependent inflammatory response. a–d C57BL/6J ( B6 ) and Myd88 −/− mice ( n = 6 each genotype) were i.p . injected with CCN1 protein (5 µg in 300 µl PBS), and peritoneal exudates were analyzed for TNFα (30 min) and IL6, KC, and MCP1 (2 h) using ELISA. e Complete blood count (CBC) analysis was performed, and neutrophils and lymphocytes contents are shown. f Gene expression induced by CCN1. BMDMs from B6 or Myd88 −/− mice were treated with CCN1 protein (2 µg per ml), LPS (50 ng per ml), or PGN (5 µg per ml) for 6 h. Tnfa and Il6 mRNAs were quantified by qRT-PCR analyses. All data are represented as mean ± s.d. acquired in triplicate determinations. Statistical evaluation was performed by one-sided, two-sample with equal variance t -tests. ** p < 0.01, and n.s. = not significant. Source data are provided as a Source Data file. Full size image The possibility that CCN1 can activate TLR signaling suggests that it may physically interact with TLRs, among which TLR2 and TLR4 are principal receptors for bacterial PAMPs and DAMPs [18] , [51] . Remarkably, we found that both human recombinant TLR2 and TLR4 proteins, which do not contain MD2, efficiently bound immobilized CCN1 in a dose-dependent manner in a solid-phase-binding assay (Fig. 8a ). CD14, an LPS transport protein, failed to show binding as a negative control, indicating specificity of the assay. Fig. 8: CCN1 binds and activates TLR2 and TLR4. a Solid-phase-binding assays between CCN1 and TLR2/4. Recombinant TLR2 or TLR4 proteins (200 ng per well) were added to 96-well plates pre-coated with serially diluted CCN1 protein at indicated amounts. Specific interaction was detected and quantified using polyclonal anti-hTLR2 or anti-hTLR4 antibodies. Recombinant CD14 (200 ng per well) was used as a control. b SPR analyses of CCN1 binding to TLR2. TLR2 was immobilized on CM5 chip and various concentrations of CCN1 was injected as analyte. c Sensorgrams of CCN1 binding to TLR4 analyzed by SPR as in b . d Dot blot analyses of CCN1 and mutant proteins binding to TLR2/4. CCN1-WT, CCN1-D125A, or CCN1-DM proteins (1 µg each) were spotted onto nitrocellulose membrane and incubated with TLR2 or TLR4 proteins (2 µg each in PBS) for 4 h. Binding was detected using polyclonal anti-hTLR2 or anti-hTLR4 antibodies. A representative image is shown. e Tnfa and Il6 mRNAs were quantified in BMDMs from either B6 or MyD88 −/− mice treated with CCN1-WT, CCN1-D125A, and CCN1-DM mutant proteins using qRT-PCR analysis. f Tnfa and Il6 mRNAs from BMDMs of B6 , Tlr2 −/− , or Tlr4 −/− mice treated with CCN1 proteins (CCN1-WT, -D125A, -DM, 2 μg per ml each) were quantified using qRT-PCR analyses. All data are represented as mean ± s.d. acquired in triplicate determinations. Statistical evaluation was performed by one-sided, two-sample with equal variance t -tests. * p < 0.05, ** p < 0.01, and n.s. = not significant. Source data are provided as a Source Data file. Full size image To further confirm the binding of CCN1 to TLR2 and TLR4 and to assess binding affinity, we performed SPR analysis (Fig. 8b, c and Supplementary Fig. 13 ). Sensorgrams showed CCN1 interacted specifically with TLR2 and TLR4 immobilized on CM5 sensor chip with K D values of 227 nM and 291 nM, respectively. In addition, SPR analysis also confirmed specific interaction between CCN1 and its phagocytic receptor, integrin α v β 3 , with a K D of 202 nM (Supplementary Fig. 13 ). These results clearly show that CCN1 binds TLR2 and TLR4 directly with affinities similar to its binding to the phagocytic receptor integrin α v β 3 . Further analysis by immunoblotting showed that CCN1-WT and CCN1-D125A bound to both TLR2 and TLR4, whereas CCN1-DM only bound TLR4 but not TLR2 (Fig. 8d ). These findings indicate that the DM mutations disrupted the CCN1-binding site for TLR2. Consistent with this binding pattern, CCN1-WT and CCN1-D125A induced a higher level of inflammatory gene expression in B6 BMDMs compared to CCN1-DM, which only bound TLR4 but not TLR2 (Fig. 8e ). Induction of Tnfa and Il6 was abolished in BMDMs from Myd88 −/− mice, consistent with CCN1 activation of TLR signaling (Fig. 8e ). To further confirm that CCN1 activates gene expression through direct binding to TLRs, we examined the effects of CCN1 in BMDMs from knockout mice deficient in TLR2 or TLR4. Induction of Tnfa and Il6 by CCN1-WT and CCN1-D125A was reduced in BMDMs of either Tlr2 −/− or Tlr4 −/− mice, indicating that CCN1 activates gene expression through both TLR2 and TLR4 (Fig. 8f ). However, CCN1-DM-induced gene expression was eliminated only in Tlr4 −/− BMDMs but unchanged in Tlr2 −/− BMDMs (Fig. 8f ), consistent with the selective binding of CCN1-DM to TLR4 but not TLR2 (Fig. 8d ). Altogether, these results show that CCN1 can directly bind and activate TLR2 and TLR4 and may function as a DAMP to regulate inflammatory responses, independent of bacterial infections. In a hostile environment replete with numerous and disparate microbial invaders, animal hosts have developed multiple arsenals for self-defense. Opsonins are structurally diverse frontline defense molecules that recognize and bind bacteria to mark them for phagocytosis and elimination through specific cell surface receptors [52] . Families of opsonins include antibodies, complement proteins, and factors such as pentraxins (serum amyloid P and C-reactive protein) [53] , [54] , collectins [55] , and ficolins [56] . As each opsonin may have idiosyncratic target specificities and efficacy, the nature and availability of specific opsonins at the sites of infection may affect the pathological outcome. Here, we show that the matricellular protein CCN1 is an opsonin for both Gram-positive and Gram-negative bacteria, including S. aureus (MRSA) and P. aeruginosa and promotes their removal by phagocytosis and ROS-mediated killing (Fig. 9 ). Ccn1 is essential for efficient bacterial clearance in mouse models of infection, and administration of CCN1 protein markedly accelerates bacterial clearance. As the emergence of antibiotic-resistant bacteria is a critical public health issue [2] , [3] , the efficacy of CCN1 against these common antibiotic-resistant pathogens suggests potential therapeutic value. Fig. 9: Schematic of CCN1 functions in bacterial clearance and activation of TLR signaling. CCN1 functions as a PRR and opsonizes Gram-positive and Gram-negative bacteria through binding PGN and LPS, respectively. CCN1 activates phagocytosis by engagement of integrin α v β 3 in phagocytes, thereby promoting the engulfment of bacteria. In macrophages, CCN1 also stimulates ROS production through activation of Rac1 and NOX2, thus enhancing bacterial killing. Independent of the presence of bacteria, CCN1 functions as a DAMP and activates TLR2 and TLR4 by direct binding to these receptors, leading to MyD88-dependent expression of inflammatory cytokines and chemokines. Full size image Our current study was predicated on the discovery that CCN1 acts as a bridging molecule for efferocytosis of apoptotic neutrophils [25] . However, most bridging molecules for efferocytosis are incapable of opsonizing bacteria, an activity that requires specific recognition of bacterial PAMPs [57] . The binding of CCN1 to PGN of S. aureus is mediated through both the vWC and TSR domains (Fig. 1c, g and Supplementary Fig. 3 ). Although thrombospondin-1 (TSP-1) has been shown to bind PGN [58] , whether this binding occurs through the TSR domain of TSP-1 is unknown. The TSR of mindin binds LPS and LTA [59] , whereas TSR of BAI1 binds only LPS [60] . In CCN1 the TSR binds PGN but not LPS (Supplementary Fig. 3 ), underscoring the functional diversity of various TSR domains. By contrast, CCN1 recognition of LPS is dependent on a cluster of positively charged residues in the CT domain (Fig. 1g ) [35] . CCN1 can also bind other bacteria, including the Gram-positive S. pneumoniae and the intracellular Gram-negative S. typhimurium (Supplementary Fig. 4 ), indicating that CCN1 may potentially opsonize a broad spectrum of bacterial species. Phagocytosis is a well-coordinated process involving target recognition and tethering, followed by engulfment of the cargo to form an intracellular membrane-enclosed phagosome [61] . CCN1 engages integrin α v β 3 as the phagocytic receptor, leading to the activation of the small GTPase Rac1 (Fig. 2 ), which is known to regulate actin cytoskeleton reorganization, cell motility, and phagocytic cup formation [62] , [63] . We have previously shown that in efferocytosis CCN1 activates Rac1 in macrophages upon engagement of integrin α v β 3 , leading to formation of the integrin-p130 Cas /CrkII complex [25] . This complex recruits DOCK180, a Rac1-activating guanine nucleotide exchange factor (GEF), thereby activating Rac1 [64] , [65] . Thus, CCN1 engagement of integrin α v β 3 and activation of Rac1 play crucial roles in the phagocytosis of both apoptotic cells and bacterial pathogens. Indeed, CCN1-induced Rac1 activation not only regulates phagocytic engulfment of bacteria but is also critical for NOX2-dependent ROS generation to eliminate ingested bacteria (Figs. 2 and 3 ), thereby parsimoniously coupling these two molecularly distinct but functionally connected events. We have employed two mouse models, Ccn1 ΔMyeloid and Ccn1 D125A/D125A mice, to provide genetic evidence for the role of CCN1 in antibacterial defense in vivo (Figs. 4 and 5 ). First, increased mortality and tissue colonization in Ccn1 ΔMyeloid mice upon S. aureus (MRSA USA300) and P. aeruginosa infection clearly demonstrate the importance of CCN1 expressed in myeloid phagocytes for efficient defense against these pathogens. Second, Ccn1 D125A/D125A knock-in mice exhibited similar defects in bacterial clearance, underscoring the critical role of CCN1 activities mediated through α v integrins, including phagocytosis and generation of bactericidal ROS (Figs. 2 and 3 ). Interestingly, some of the distinct phenotypes of these two mouse models also hinted at cell type- and integrin-specific CCN1 functions (Figs. 4d and 5c ). For example, the formation of pyogenic abscesses was prominent only in Ccn1 ΔMyeloid mice but not in Ccn1 D125A/D125A mice, suggesting that myeloid cells-derived CCN1 may have negative effects on abscess formation through α v -independent pathways, possibly by regulating bacterial proteins important for abscess formation such as coagulase (Coa) and vWbp [66] , [67] . By contrast, the Ccn1 D125A/D125A knock-in mice showed shrunken glomeruli and convoluted tubules of the renal cortex area upon S. aureus infection (Fig. 5c ), suggesting that integrin α v -mediated CCN1 functions in parenchymal tissues may be critical for injury repair [68] . Consistent with a role for CCN1 in parenchymal repair, CCN1 has been shown to be essential for the regeneration of bile ducts [27] and the intestinal epithelium [28] after injuries. In cutaneous wound healing, CCN1 promotes the removal of apoptotic neutrophils, accelerates wound healing progression [25] , and promotes matrix remodeling [26] . The ability of CCN1 to enhance bacterial clearance may contribute to the healing of wounds at risk of infections. In this regard, S. aureus and P. aeruginosa are the two most commonly found bacterial pathogens in chronic wounds such as diabetic wounds [69] , [70] . To our surprise, we found that CCN1 can by itself induce inflammatory responses in the absence of bacterial infection through physical interaction with TLR2 and TLR4 to activate MyD88-dependent signaling (Figs. 7 and 8 ). These findings suggest that CCN1 may act as an alarmin or DAMP to trigger sterile inflammation upon tissue injury to initiate repair. SPR analysis showed that CCN1 binds TLR2 and TLR4 with K D values of 227 nM and 291 nM, respectively. This binding is somewhat stronger than the interaction of HMGB1, a well-characterized DAMP, with the TLR4/MD2 complex ( K D = 420 nM) or TLR4 alone ( K D = 650 nM) [71] . Since CCN1 is released from platelet α-granules upon platelet activation [72] , which is triggered by vascular damage, it can be rapidly available upon injury to induce sterile inflammation and tissue repair through direct binding to TLRs. Deregulation of CCN1 may contribute to inflammatory pathologies, as CCN1 has been associated with chronic inflammatory diseases, including rheumatoid arthritis [73] , atherosclerosis [74] , diabetic nephropathy and retinopathy [75] , [76] , and inflammation-related cancers [29] , and targeting CCN1 with antibodies or siRNAs ameliorates disease symptoms in animal models of rheumatoid arthritis and diabetic retinopathy [73] , [76] . As several previous reports on TLR-activating proteins have been confounded by the potential presence of PAMPs in the reagents used [51] , we have reinforced our findings through several lines of evidence. First, our CCN1 proteins were expressed in mycoplasma-free insect cells rather than from bacterial sources. The presence of LPS was not >0.08 EU (8 pg) per µg CCN1 as judged by the Limulus Amebocyte Lysate (LAL) assay (Supplementary Fig. 14 ), below the amount necessary to elicit a minimal discernible induction of cytokine expression in various cell types [77] . Further purification through a polymyxin-B column to remove any residual endotoxin did not change its inflammation-inducing activity (Supplementary Fig. 14 ). Second, the CCN1-DM mutant is unable to bind LPS, yet it can bind TLR4 and induce TLR4 signaling (Figs. 1 g and 8f ), indicating CCN1 activation of TLR is independent of LPS binding. Further, CCN1-DM is defective for binding TLR2 and is correspondingly unable to induce TLR2 signaling, indicating that TLR binding and activation require specific sequences in the CCN1 polypeptide (Fig. 8d, f ). Finally, genetic evidence from Ccn1 ΔMyeloid and Myd88 −/− mice showed that CCN1 contributes to inflammatory responses through MyD88, supporting its functions through TLRs in vivo (Figs. 6 and 7 ). Altogether, these observations provide compelling evidence that CCN1 acts as a TLR-activating DAMP. S. aureus and P. aeruginosa have developed diverse mechanisms of immune evasion by interfering with host opsonins, particularly those that are constitutively expressed [78] , [79] . For example, mucoid exopolysaccharides from P. aeruginosa interferes with complement-dependent phagocytosis [80] , and protein A of S. aureus binds to the Fc region of IgG, thereby blocking FcR-dependent phagocytosis [81] , [82] . However, it appears that neither S. aureus nor P. aeruginosa has the ability to counteract the opsonin activities of CCN1, as demonstrated by results in Ccn1 genetic models and the clear efficacy of exogenous CCN1 in promoting clearance of these bacteria (Figs. 4 and 5 , and Supplementary Fig. 10 ). Furthermore, the activity of CCN1 as an opsonin should be indifferent to the antibiotic resistance status of the bacterial strains. Thus, CCN1 may potentially be useful therapeutically against a broad range of Gram-positive and Gram-negative antibiotics-resistant bacteria. Further studies that define the minimal functional domains of CCN1 for opsonization and phagocytosis may allow the construction of peptides that link these domains for bacterial clearance. Future investigation into the potential efficacy of CCN1 and CCN1-derived peptides may prompt novel therapies for bacterial infections recalcitrant to conventional treatments. CCN1 proteins and reagents Recombinant CCN1 and mutant proteins (CCN1-D125A, CCN1-DM, CCN1-ΔCT, and IGFBP-vWC; Supplementary Fig. 1 ) were produced using a baculovirus expression system in Sf9 insect cells and purified by ion-exchange or immuno-affinity chromatography [34] , [36] . Sf9 cells were routinely tested for mycoplasma contamination using LookOut ® Mycoplasma PCR detection kit (Sigma, MP0035). CCN1 preparations were tested for the presence of LPS using Limulus Amebocyte Lysate (LAL) Chromogenic Endotoxin Quantification kit (Thermo Scientific, 88282) and found not >0.08 EU per μg CCN1 (Supplementary Fig. 14A ). Further purifications through a polymyxin-B-agarose column (Sigma, P1411; 1 mg per ml; binding capacity of 200–500 µg LPS per 1 mg) to remove any endotoxin did not eliminate CCN1 (Supplementary Fig. 14B ). Individual CCN1 domain fragments (IGFBP, vWC, TSR) were produced as GST-fusion proteins and purified using a glutathione-Sepharose column [83] . Additionally, CCN1 proteins were purchased from R&D biosystems (4055-CR-050) and Novus (NBP2-34944) to test CCN1 activities (Supplementary Fig. 14 ). Rabbit and goat IgGs were purchased from Fisher Scientific. LPS (L9143) from P. aeruginosa , PGN (77140) and LTA (L2515) from S. aureus , Rac1 inhibitor (NSC23766; 553502), PI3K inhibitor (LY294002; 19-142), ERK inhibitor (PD98059; 19-143), p38 MAPK inhibitor (SB203580; S8307), cytochalasin D (C2618), and Apocynin (178385) were from Sigma. NOX1 inhibitor (ML-171; 492002) was from EMD Millipore. NOX2 inhibitor (GSK2795039; HY-18950) was from MedChemExpress. Cilengitide (S7707) was from SellecChem. Bacterial culture All bacterial stains used were obtained from ATCC. Methicillin-resistant S. aureus strain USA300 (ATCC®-BA1717™), P. aeruginosa (ATCC®-27107™), S. pneumoniae (ATCC®-6303™), and S. typhimurium (ATCC®-14028™). S. aureus and P. aeruginosa were cultured overnight in tryptic soy broths, diluted at 1:100 and grown exponentially. In general, OD A600 = 1 corresponded to 1.5 × 10 9 CFU per ml for S. aureus and 7.5 × 10 8 CFU per ml for P. aeruginosa . Bacteria were used at their exponential growth phase (OD A600 = ~0.6). S. pneumoniae and S. typhimurium were grown in Brain-Heart infusion broth (Sigma, 53286). Animals and bacterial infection models Animal protocols were approved by the Institutional Animal Care and Use Committee of The University of Illinois at Chicago (ACC#17-001). Ccn1 D125A/D125A and Ccn1 DM/DM knock-in mice [25] , [26] were generated in a svJ129-C57BL/6J mixed background and backcrossed to the C57BL/6J strain 6 and 11 times, respectively. Ccn1 ΔMyeloid mice were generated by crossing Ccn1 flox/flox with myeloid-specific Cre deleter stain, LysM-Cre (B6.129P2- Lyz2 tm1(cre)Ifo /J, 004781). Tlr2 −/− (B6.129- Tlr2 tm1Kir /J, 004650), Tlr4 −/− (B6(Cg)- Tlr4 tm1.2Karp /J, 029015), and Myd88 −/− mice (B6.129P2(SJL)- Myd88 tm1.1Defr /J,009088) were from the Jackson Laboratory. All mice were housed in sterile static microisolator cages on autoclaved corncob bedding with water bottles. Both irradiated food and autoclaved water were provided ad libitum. The standard photoperiod was 14 h of light and 10 h of darkness. Mice (both male and female) at 10–12 weeks of age with similar body weight (25–28 g) were used in bacterial infection studies. For bacteremia and tissue colonization studies, mice were anesthetized by intraperitoneal ( i.p .) injection of ketamine (100 mg per kg) and xylazine (10 mg per kg) and systemically infected with S. aureus (7.5 × 10 8 CFU per mouse for survival, 2 × 10 8 CFU per mouse for tissue colonization) through retro-orbital delivery. Liver (whole-left lateral lobe), kidney (two whole-organs per mouse) and the whole heart were harvested and processed for bacterial colonization and histological analyses. For acute peritonitis model, mice were infected by i.p . injection of S. aureus (5 × 10 7 CFU per mouse) or P. aeruginosa (5 × 10 7 CFU per mouse) and peritoneal exudate or whole blood were examined for bacterial blood dissemination and cytokines/chemokines production. In CCN1 protein injection studies, purified CCN1 (5 µg in PBS) was i.p . injected in animals to analyze inflammatory responses or injected 1 h after S. aureus infection to monitor bacterial clearance. For skin and soft-tissue infection (SSTI), a bolus of S. aureus (4 × 10 6 CFU per mouse) was subcutaneously injected into mouse flank skin and blood dissemination was monitored. Complete blood count Mice with acute peritonitis had total blood drawn via cardiac puncture and complete blood count (CBC) was analyzed using Advia 120 analyzer (Siemens). Cell culture and isolation All cell lines were obtained from ATCC. L-929 cells (ATCC®CCL-1™) were grown in Dulbecco's modified Eagle medium (DMEM) Glutamax I media (Invitrogen) supplemented with 10% (vol per vol) heat-inactivated fetal bovine serum (FBS, Hyclone™), 1% HEPES, and 1% penicillin-streptomycin (Invitrogen) in a humidified incubator with 5% CO 2 at 37 °C. For preparation of conditioned medium, L-929 cells were plated at density of 4.7 × 10 5 cells in a 75-cm 2 flask containing 55 ml culture medium and grown for 7 days. Collected supernatant was filtered through a 0.45 µm filter and stored at –30 °C. THP.1 cells (ATCC®TIB-202™) were grown in suspension in RPMI Glutamax media (Invitrogen) supplemented with 10% FBS and 0.05 mM β-mercaptoethanol. For differentiation, THP.1 cells at low passage (<15) were plated in 4-well chamber slide in the presence of phorbol-12-myristate-13-acetate (PMA, 100 nM; Sigma) for 3 days. Peritoneal macrophages were isolated from peritoneal exudates of mice elicited with thioglycolate (3% vol per weight) for 3 days [84] . Bone marrow-derived neutrophils (PMNs) were isolated by differential centrifugation [25] . The purity of the neutrophil fraction was assessed by Giemsa staining (Sigma); over 99% purity was typically obtained. For BMDMs, the total bone-marrow cells were re-suspended in macrophage complete media (DMEM/F12 with 10% FBS and 20% L-929 cells conditioned media), and 4 × 10 5 cells were plated in sterile plastic petri dish (100 mm) and incubated in 5% CO 2 at 37 °C for 7 days with medium being refreshed every 3 days for differentiation into macrophages. Macrophage differentiation was assessed by F4/80 immunostaining; typically, over 90% are F4/80 positive. For splenic B or T cells isolation, total spleen was excised and homogenized between frosted ends of microscope slides in Hank’s Balanced Salt Solution. Subsequently, B or T cells were isolated using Nylon Wool Fiber Columns (Polysciences) according to manufacturer’s instruction. Bacterial phagocytosis and killing For S. aureus phagocytosis, BMDMs were labeled with CellTracker™ Green-CMFDA (5-chloromethylfluorescein diacetate) fluorescent dye (5 µM, Invitrogen) for 30 min. Cells were either untreated or pretreated with CCN1 proteins (CCN1-WT, -D125A, and -DM; 2 µg per ml each) for 1 h, followed by incubation with S. aureus bioparticle (pHrodo® Red S. aureus BioParticles™ conjugates; Invitrogen, 5 µg per ml) for an additional 45 min. Cells were washed with ice-cold PBS five times and fixed with paraformaldehyde (4% vol per vol in PBS). Images were taken using fluorescence microscopy (Leica DM4000B). Phagocytosis was quantified by counting macrophages containing >2 S. aureus particles in 12 randomly selected high-powered fields and expressed as a percentage of positive macrophages over total cells counted (~300 cells). For all inhibitor experiments, cells were pretreated with chemical inhibitors for 30 min prior to CCN1 treatment. To monitor bacterial killing after phagocytosis, BMDMs were allowed to phagocytose S. aureus (MOI of 10) for 90 min, followed by CCN1 treatment with or without chemical inhibitors. To remove unphagocytosed S. aureus , lysostaphin (10 µg per ml; Sigma) was added for 15 min. Cells were lysed in Triton X-100 (0.04% vol per vol) and plated with serial dilution on tryptic soy agar plates with 5% sheep blood for bacterial enumeration. To monitor phagocytosis of P. aeruginosa , BMDMs were pretreated with CCN1 proteins, followed by incubation with P. aeruginosa (MOI of 10) for 45 min. Cells were treated with gentamycin (200 µg per ml; Gibco) for 15 min to eliminate extracellular or membrane-bound bacteria, lysed in Triton X-100 (0.04% vol per vol), and plated with serial dilution on tryptic soy agar with 5% sheep blood for bacterial enumeration. ROS measurement For measurement of superoxide radicals ( O 2 − ), BMDMs were grown in 4-well chamber slides and pre-loaded with dihydroethidium (DHE, 5 µM; Invitrogen) in serum-free media for 1 h. Cells were then treated with CCN1 proteins in full growth media for an additional 45 min and washed with ice-cold PBS three times. High-resolution images were taken from randomly selected fields using fluorescence microscopy (Leica DM4000B) and fluorescence intensity of individual cells (>50 cells) was analyzed using Image J (NIH). Chemical inhibitors were treated 30 min prior to CCN1 proteins. Cells were kept in darkness during the entire procedure. Solid-phase-binding assay and dot blot analysis The physical interaction of CCN1 with bacteria ( S. aureus or P. aeruginosa ) or TLRs was analyzed in solid-phase-binding assays. Ninety-six-well plates were coated with serially diluted CCN1 or other ECM proteins in bicarbonate/carbonate coating buffer (100 mM, pH 9.6) overnight at 4 °C. After washing three times with PBS-Tween20 (PBST), plates were then blocked with poly-vinyl alcohol (PVA, 2% vol per weight) for 1 h. For bacterial binding, S. aureus or P. aeruginosa (8 × 10 3 CFU per well in 100 µl PBS) was added to each well and incubated for 1 h. After washing with PBST three times, bound bacteria were detected using polyclonal anti- S. aureus (abcam, ab20920; 1:2000 dilution) or anti- P. aeruginosa antibodies (abcam, ab69232; 1:500 dilution), visualized with horseradish peroxidase (HRP)-conjugated secondary antibodies with 3,3′,5,5′- Tetramethylbenzidine (TMB) as a substrate, and quantified in a microplate reader (Labsystems Multiskan MS) at A450 nm. Absorbance at A570 nm was used to correct for minor optical imperfections of plates. All assays were done in triplicates and in three independent experiments. For TLRs interaction, hTLR2, hTLR4, or hCD14 (0.2 µg per well, R&D systems) were incubated with coated CCN1 proteins and detected using polyclonal anti-hTLR2 (AF2616), anti-hTLR4 (AF1478), or monoclonal anti-hCD14 antibodies (MAB3832, R&D systems; 1:100 dilution each,) as described above. In some cases, interactions were assayed in dot blot analyses. Briefly, bacterial pattern molecules (PGN, LTA, or LPS; 1 µg each) were spotted on nitrocellulose membranes and air-dried for 30 min. Each membrane was incubated with CCN1 proteins (CCN1-WT, -D125A, or -DM proteins; 5 µg  in 5 ml PBS each) and bound CCN1 was detected with polyclonal anti-CCN1 antibodies (1:2000 dilution) using chemiluminescence. For TLRs binding, CCN1 proteins (CCN1-WT, -D125A, and -DM; 1 µg each) were spotted, followed by incubation with hTLR2 or hTLR4 (each 5 µg  in 5 ml PBS). Bound TLRs were detected with polyclonal anti-hTLR2 or anti-hTLR4 antibodies (1:1000 dilution each). Flow cytometry S. aureus collected in the logarithmic phase were heat-killed in 80 °C for 30 min and re-suspended in PBS buffer containing 2 mM EDTA and 0.5% BSA. S. aureus (10 8 CFU per ml) were then incubated with increasing concentrations of either CCN1 or recombinant human C3b complement proteins (Sigma, 204860) for 1 h at room temperature. After washing once with buffer, rabbit polyclonal anti-CCN1 antibody (1:100 dilution) or mouse monoclonal anti-iC3b antibody (EMD Millipore, MABF972; 1:200 dilution) were added for 1 h, followed by allophycocyanin (APC)-conjugated goat anti-rabbit IgGs (Life Technologies Co.; A10931, 1:250 dilution;) or APC-conjugated rat anti-mouse IgGs (Life Technologies Co.; 17-4015-82, 1:500 dilution), respectively. S. aureus was then analyzed using CytoFLEX S flow cytometer (APC channel, Beckman Coulter) and histograms were generated using CytoExpert software. The gating strategy is shown in Supplementary Fig. 2 . SPR analysis SPR studies were performed using a Biacore T-200 (Biacore Inc., GE Healthcare) biosensor system according to the manufacturer’s instructions. TLR2, TLR4 and integrin α v β 3 proteins were directly immobilized on a CM5 sensor chip using the standard amine-coupling method. The carboxymethylated dextran surface was activated by 1-ethyl-3-(3-dimethylaminoprophyl) carbodiimide hydrochloride (EDC)/N-hydroxy succinimide (NHS) mixture. TLR2 (2616-TR-050, R&D systems), TLR4 (1478-TR-050) and integrin α v β 3 proteins (3050-AV-050) were diluted with 10 mM sodium acetate buffers (pH 4.0) and immobilized on respective flow channels, followed by ethanolamine blocking of the unoccupied surface area. As an analyte, various concentrations of CCN1 were applied at 25 µl per min flow rate at 25 °C  in phosphate buffer containing 350 mM sodium chloride, 0.5 mM calcium chloride and 0.5 mM magnesium chloride and 10 µg per ml BSA. LPS was immobilized on a hydrophobic HPA sensor chip and CCN1 protein was used as analyte. For immobilization, the HPA surface was washed with a 5-min injection of 40 mM octyl glucoside in water, followed by LPS injection at a low flow rate (5 µl per min). Loosely bound LPS was then removed by washing the surface with a short injection (1 min) of 100 mM sodium hydroxide. The instrument was kept completely detergent-free and buffers were thoroughly degassed for experiment with HPA chip as recommended. Data (response unit, RU) were double subtracted by blank reference channel and zero concentration analyte signal. Sensorgrams were analyzed using the Biacore T-200 evaluation software V.3.0 and kinetic rate constants ( k a and k d ) were determined by fitting globally to the 1:1 Langmuir (one-to-one binding) model embedded within the software. The equilibrium dissociation constant ( K D ) was calculated as the ratio of these two constants ( k d / k a ). Tissue histology Liver and kidney tissues from mice at 5 day post infection were snap-frozen in optimum cutting temperature (OCT) compound (Tissue-Tek) and sectioned serially (7 μm) using a Leica CM1950 UV cryostat. Sections fixed with cold acetone were stained with Hematoxylin/Eosin (H&E) or probed with polyclonal anti- S. aureus antibodies (abcam; ab20920, 1:100 dilution) in immunofluorescence staining using Alexafluor488-conjugated anti-rabbit IgG (Invitrogen, 1:500 dilution). DAPI was used as the counterstain (1 mg per ml, Sigma). Fluorescence images were acquired using a Leica DM4000B microscope and processed with Photoshop CC 2019 (Adobe). Knockdown of integrin subunit in BMDMs Predesigned Dicer-Substrate Short Interfering RNAs (DsiRNAs, 2 nM; Integrated DNA Technologies) against specific integrin subunits were transfected into BMDMs using SuperFect Transfection reagent (Qiagen) according to manufacturer’s manuals. 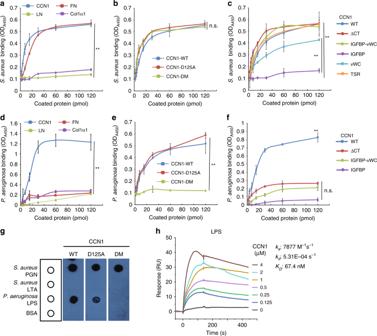Fig. 1: CCN1 bindsS. aureusandP. aeruginosathrough PGN and LPS, respectively. CCN1 binding toS. aureus(a–c) andP. aeruginosa(d–f) was evaluated using a solid-phase-binding assay.aS. aureusbound to surfaces coated with CCN1-WT or other ECM proteins (FN fibronectin, LN laminin, Col1α1 collagen type I) was quantified using polyclonal anti-S. aureusantibodies. CCN1 and FN bound toS. aureus, whereas LN and Col1α1did not.bBinding assay ofS. aureusto recombinant CCN1-WT, CCN1-D125A, and CCN1-DM proteins as above.cBinding ofS. aureusto CCN1 deletion mutant proteins as above.dSolid-phase-binding assays forP. aeruginosawere performed as above and detected with polyclonal anti-P. aeruginosaantibodies.eBinding assay showingP. aeruginosabinding to CCN1-WT and CCN1-D125A, but not CCN1-DM.fSolid-phase-binding assays with CCN1 deletion mutants. All assays were done in triplicates and data are expressed as mean ± s.d. Statistical evaluation was performed by one-sided, two-sample with equal variancet-tests. **p< 0.01, n.s. = not significant.gBacterial molecular patterns (PGN ofS. aureus; LTA ofS. aureus; LPS ofP. aeruginosa; 1 µg each) and BSA as control spotted on nitrocellulose membranes were incubated with CCN1 proteins (WT, D125A, or DM; 2 µg each in PBS) and bound CCN1 was visualized using anti-CCN1 antibodies. Dot blot shown is a representative image.hSenograms of SPR analysis of CCN1 binding to LPS. CCN1 at various concentrations was used as analyte to detect binding to LPS immobilized on HPA hydrophobic sensor chip.Ka,Kd, andKDvalues were obtained by kinetic analysis. Knockdown efficiencies (>90%) were confirmed using quantitative reverse transcription PCR (qRT-PCR) analyses after 24 h. DsiRNA sequences used for knockdown are shown in Supplementary Table 1. Quantification of cytokines and chemokines Mice were challenged with acute peritonitis induced by either S. aureus infection or CCN1 injection. Peritoneal exudates were harvested with 4 ml ice-cold PBS using 18-gauge needles; cytokines and chemokines were quantified using ELISA kits: mTNFα (88-7324-22, eBioscience), mIL6 (88-7064-22, eBioscience), KC (EMCXCL1, Invitrogen), and mMCP-1 (88-7391-22, Fisher Scientific). RNA isolation and qRT-PCR Cultured BMDMs were homogenized using TRIzol reagent (Invitrogen) and total RNAs were purified using RNeasy® Mini Kit (Qiagen). 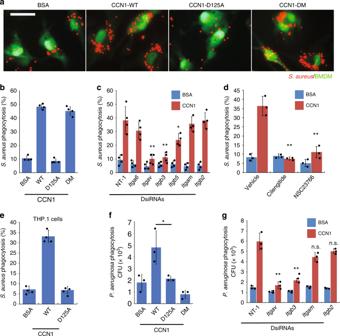Fig. 2: CCN1 stimulates phagocytosis of bacteria through αvintegrins in macrophages. BMDMs (labeled with CellTrackerTMGreen) were pretreated with either BSA, CCN1-WT, CCN1-D125A, or CCN1-DM proteins (2 µg per ml) followed by incubation with bacteria for 45 min.aPhagocytosis ofS. aureus(pHrodo Red conjugates) is shown in representative images from fluorescence microscopy. Scale bar = 40 µm.bQuantification of phagocytosis ofS. aureusby BMDMs pretreated with various proteins.cBMDMs were transfected with DsiRNAs to knockdown integrins α6, αv, β3, β5, αM, or β2; knockdown efficiencies are shown in Supplementary Fig.6. Cells were then pretreated with CCN1 or BSA, and phagocytosis ofS. aureuswas quantified. NT-1, non-targeting RNA.dEffect of cilengitide (1 µM) and the Rac1 inhibitor NSC23766 (10 µM) on CCN1-induced phagocytosis ofS. aureus.eCCN1-induced phagocytosis in differentiated THP.1 human macrophages.fBMDMs were pretreated as above and then incubated with liveP. aeruginosa(MOI of 10) for 45 min, followed by gentamycin (200 µg per ml for 15 min) treatment. Phagocytosis was measured by enumeration of bacterial colonies grown from cell lysates.gEffects of DsiRNA-mediated knockdown of integrins αv, β3, αM, or β2on CCN1-induced phagocytosis ofP. aeruginosa. All data are expressed as mean ± s.d. in triplicate determinations. Statistical evaluation was performed by one-sided, two-sample with equal variancet-tests. *p< 0.05, **p< 0.01, n.s. = not significant. Source data are provided as a Source Data file. Total RNAs (2 μg) were reverse transcribed to complementary DNA using MMLV-Reverse Transcriptase (Promega), and qRT-PCR was performed with the iCycler Thermal Cycler (Bio-Rad) using iQ SYBR Green Supermix (Bio-Rad). The specificity of qRT-PCR was confirmed by agarose gel electrophoresis and melting curve analysis. A housekeeping gene ( Cyclophilin E ) was used as an internal control. The primers used are following: Tnfa , forward 5′-CATCTTCTCAAAATTCGAGTGACAA-3′, reverse 5′-TGGGAGTAGACAAGGTACAACCC-3′; Il6 , forward 5-GAGGATACCACTCCCAACGAGCC-3′, reverse 5′-AAGTGCATCATCGTTGTTCATACA-3′; Cyclophilin E ( CypE ), forward 5′-TTCACAAACCACAATGGCACAGGG-3′, reverse 5′-TGCCGTCCAGCCAATCTGTCTTAT-3′. Statistics All experimental results are expressed either as mean ± standard deviation (s.d.) 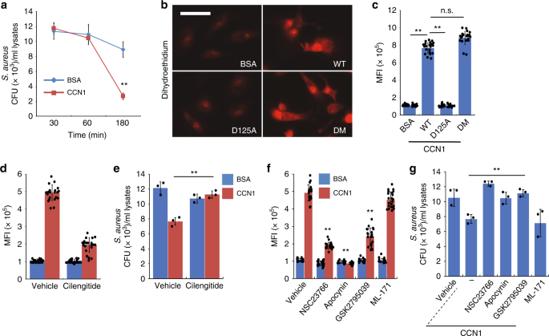Fig. 3: CCN1 enhances bacterial killing after phagocytosis through ROS production. aLysostaphin protection assay for assessingS. aureuskilling after phagocytosis. After BMDMs phagocytosedS. aureusand extracellular bacteria were eliminated by lysostaphin, cells were treated with CCN1 or BSA (2 μg per ml each) and viable bacteria inside BMDMs were enumerated at indicated chase periods.bSuperoxide (O2−) was measured by dihydroethidium (DHE, 5 µM) staining in BMDMs treated with recombinant CCN1 proteins (WT, D125A, or DM; 2 µg per ml each) for 30 min. Representative images shown were acquired from fluorescence microscopy. Bar = 40 µm.cHigh-magnification images were taken from at least ten random fields and mean fluorescence intensity (MFI) was calculated using Image J software.dROS production was quantified as MFI using DHE fluorescence in BMDMs pretreated with cilengitide (1 μM), followed by CCN1 or BSA (2 µg per ml each).eS. aureuskilling assays were performed as inawith cilengitide pretreatment.fThe effects of various inhibitors on CCN1-induced ROS production. All inhibitors were added 30 min prior to CCN1 treatment. Rac1 inhibitor NSC23766 (10 µM); NOX inhibitor Apocynin (10 µM); NOX2 inhibitor GSK2795039 (10 µM); NOX1 inhibitor ML-171 (10 µM).gEffects of various inhibitors on bacterial killing using lysostaphin protection assays as above. All data were acquired from at least three independent assays and are expressed as mean ± s.d. in triplicate determinations. Statistical evaluation was performed by one-sided, two-sample with equal variancet-tests. **p< 0.01, n.s. = not significant. Source data are provided as a Source Data file. or mean with individual quantitative values in dot plots. Wherever necessary, statistical evaluation was performed by one-sided, two-sample with equal variance t -tests. 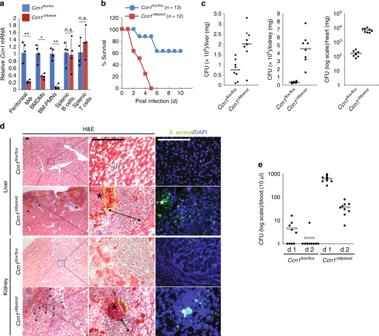Fig. 4:Ccn1expression in myeloid cells is critical for host defense againstS. aureusinfections. aCcn1mRNA in peritoneal macrophages (MΦ), BMDMs and PMNs, and splenic B and T cells fromCcn1flox/floxandCcn1ΔMyeloidmice was analyzed using qRT-PCR. Myeloid-specific deletion was confirmed using splenic B and T cells as controls. Data are represented as mean ± s.d. from triplicate experiments. Statistical evaluation was performed by one-sided, two-sample with equal variancet-tests. *p< 0.05, **p< 0.01, n.s. = not significant.bSurvival ofCcn1flox/flox(n= 13) andCcn1ΔMyeloid(n= 12) mice after infection withS. aureus(7.5 × 108CFU per mouse,i.v.).cTissue colonization ofS. aureusinCcn1flox/floxandCcn1ΔMyeloidmice infected withS. aureus(2 × 108CFU per mouse,i.v.). Bacterial counts in liver, kidney, and heart (n= 8 each) 5 days post infection were evaluated by growth of serially diluted tissue homogenates on tryptic soy agar with 5% sheep blood and plotted as CFU per mg tissues.dHistological examination of liver and kidney ofCcn1flox/floxandCcn1ΔMyeloidmice at day 5-post infection. Representative images are shown. H&E staining showed the presence of pyogenic abscesses (arrowheads in left panels) in both liver and kidney fromCcn1ΔMyeloidmice, whereas no pyogenic abscesses were found inCcn1flox/floxmice. Boxed regions with dotted line are expanded in high magnification in middle panels. Asterisk (*) points to nidus, yellow rectangular box indicates pseudo-capsule, and bidirectional arrow shows regions of neutrophils.S. aureuscolonization was visualized in adjacent sections using anti-S. aureusantibodies (green, Alexafluor488-anti-rabbit IgG) in immunofluorescence staining (right panels). DAPI (blue) was used as a counterstaining. Scale bar = 100 μm.eBlood dissemination ofS. aureuswas determined at indicated days after subcutaneous infection ofS. aureus(5 × 105CFU in 50 µl PBS) inCcn1flox/floxandCcn1ΔMyeloidmice (n= 9 each). Blood (10 µl) was plated for colony quantification. Source data are provided as a Source Data file. A p < 0.05 value was considered significant. 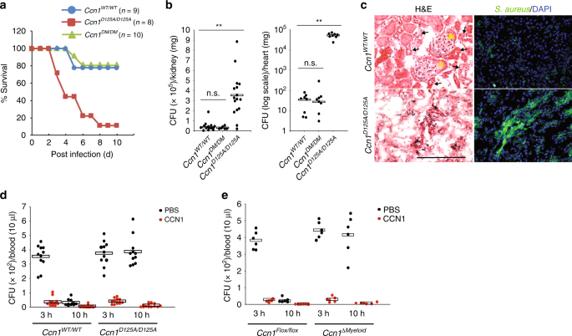Fig. 5: CCN1 functions mediated through its integrin αv-binding site are crucial for host defense. aSurvival was monitored in mice infected withS. aureus(7.5 × 108CFU per mouse,i.v.).Ccn1WT/WT,n= 9;Ccn1D125A/D125A,n= 8;Ccn1DM/DM,n= 10.bColonization in the kidney and heart was evaluated in mice infected withS. aureus(2.5 × 108CFU per mouse,i.v.). Bacterial loads were enumerated by serial dilution of tissue homogenates at day 5-post infection inCcn1WT/WT(n= 16 for kidney,n=  8 for heart),Ccn1D125A/D125A(n= 16 for kidney,n= 8 for heart), andCcn1DM/DM(n= 6 for kidney,n= 8 for heart) mice. Statistical evaluation was performed by one-sided, two-sample with equal variancet-tests. **p< 0.01; n.s. = not significant.cHistological evaluation of the kidney cortex afterS. aureusinfection. Kidney sections fromCcn1WT/WTandCcn1D125A/D125Amice at day 5-post infection were stained with H&E. Glomeruli (yellow arrowheads) and tubules (black arrows) are intact inCcn1WT/WTmice, but severely damaged inCcn1D125A/D125Amice. Adjacent sections were visualized in immunofluorescence staining with polyclonal anti-S. aureusantibody (green) and counterstained with DAPI (blue). Scale bar = 100 µm.dTreatment of mice with CCN1 protein accelerated bacterial clearance.Ccn1WT/WTandCcn1D125A/D125Amice (n= 11 per group per genotype) were challenged with acute peritonitis by infection ofS. aureus(2 × 107CFU per mouse,i.p.), followed byi.p. injection of CCN1 protein (5 µg per mouse) or PBS 1 h-post infection. Total blood was drawn at indicated times and 10 µl was plated for colony enumeration.eCcn1flox/floxandCcn1ΔMyeloidmice (n= 6 per group per genotype) were infected withS. aureusand bacterial clearance with or without CCN1 treatment was evaluated as above. Source data are provided as a Source Data file. All quantitative experiments were performed in triplicates unless otherwise indicated. 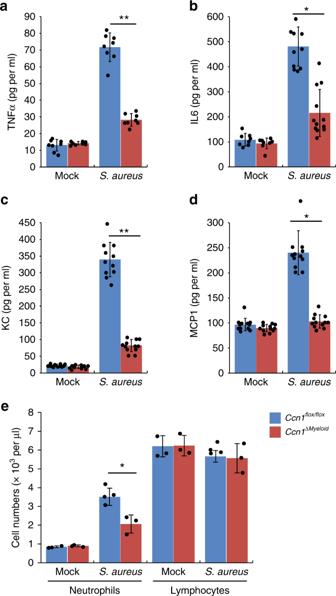Fig. 6: CCN1 is critical for the host inflammatory response upon bacterial infection. a–dQuantification of cytokines and chemokines in the peritoneum inCcn1flox/floxorCcn1ΔMyeloidmice (n= 6 per group per genotype) infected withS. aureus(2 × 107CFU per mousei.p.). Peritoneal exudates were analyzed by ELISA to quantify the levels of TNFα (a) at 30 min and IL6 (b), KC (c), and MCP1 (d) at 2 h post infection.eNeutrophils and lymphocytes contents in blood drawn at 2 h post infection were determined using Advia 120 analyzer. All data are represented as mean ± s.d. acquired in triplicate determinations. Statistical evaluation was performed by one-sided, two-sample with equal variancet-tests. *p< 0.05, **p< 0.01. Source data are provided as a Source Data file. 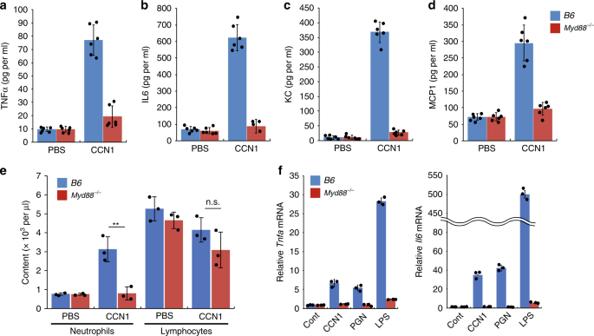Fig. 7: CCN1 inducesMyd88-dependent inflammatory response. a–dC57BL/6J (B6) andMyd88−/−mice (n= 6 each genotype) werei.p. injected with CCN1 protein (5 µg in 300 µl PBS), and peritoneal exudates were analyzed for TNFα (30 min) and IL6, KC, and MCP1 (2 h) using ELISA.eComplete blood count (CBC) analysis was performed, and neutrophils and lymphocytes contents are shown.fGene expression induced by CCN1. BMDMs fromB6orMyd88−/−mice were treated with CCN1 protein (2 µg per ml), LPS (50 ng per ml), or PGN (5 µg per ml) for 6 h.Tnfa and Il6mRNAs were quantified by qRT-PCR analyses. All data are represented as mean ± s.d. acquired in triplicate determinations. Statistical evaluation was performed by one-sided, two-sample with equal variancet-tests. **p< 0.01, and n.s. = not significant. Source data are provided as a Source Data file. 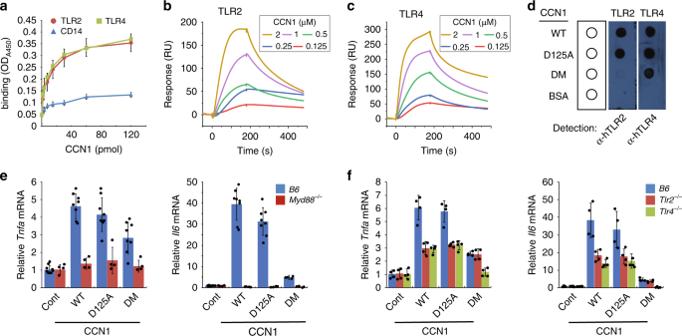Fig. 8: CCN1 binds and activates TLR2 and TLR4. aSolid-phase-binding assays between CCN1 and TLR2/4. Recombinant TLR2 or TLR4 proteins (200 ng per well) were added to 96-well plates pre-coated with serially diluted CCN1 protein at indicated amounts. Specific interaction was detected and quantified using polyclonal anti-hTLR2 or anti-hTLR4 antibodies. Recombinant CD14 (200 ng per well) was used as a control.bSPR analyses of CCN1 binding to TLR2. TLR2 was immobilized on CM5 chip and various concentrations of CCN1 was injected as analyte.cSensorgrams of CCN1 binding to TLR4 analyzed by SPR as inb.dDot blot analyses of CCN1 and mutant proteins binding to TLR2/4. CCN1-WT, CCN1-D125A, or CCN1-DM proteins (1 µg each) were spotted onto nitrocellulose membrane and incubated with TLR2 or TLR4 proteins (2 µg each in PBS) for 4 h. Binding was detected using polyclonal anti-hTLR2 or anti-hTLR4 antibodies. A representative image is shown.eTnfaandIl6mRNAs were quantified in BMDMs from eitherB6orMyD88−/−mice treated with CCN1-WT, CCN1-D125A, and CCN1-DM mutant proteins using qRT-PCR analysis.fTnfaandIl6mRNAs from BMDMs ofB6,Tlr2−/−, orTlr4−/−mice treated with CCN1 proteins (CCN1-WT, -D125A, -DM, 2 μg per ml each) were quantified using qRT-PCR analyses. All data are represented as mean ± s.d. acquired in triplicate determinations. Statistical evaluation was performed by one-sided, two-sample with equal variancet-tests. *p< 0.05, **p< 0.01, and n.s. = not significant. Source data are provided as a Source Data file. 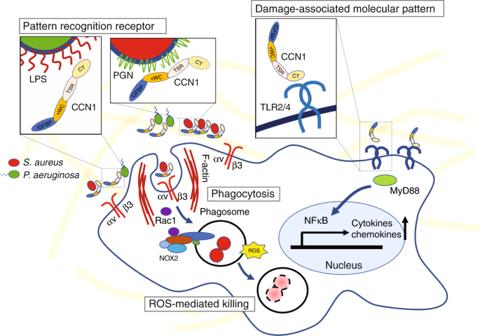Fig. 9: Schematic of CCN1 functions in bacterial clearance and activation of TLR signaling. CCN1 functions as a PRR and opsonizes Gram-positive and Gram-negative bacteria through binding PGN and LPS, respectively. CCN1 activates phagocytosis by engagement of integrin αvβ3in phagocytes, thereby promoting the engulfment of bacteria. In macrophages, CCN1 also stimulates ROS production through activation of Rac1 and NOX2, thus enhancing bacterial killing. Independent of the presence of bacteria, CCN1 functions as a DAMP and activates TLR2 and TLR4 by direct binding to these receptors, leading to MyD88-dependent expression of inflammatory cytokines and chemokines. Reporting summary Further information on research design is available in the Nature Research Reporting Summary linked to this article.